Prelamin A causes progeria through cell-extrinsic mechanisms and prevents cancer invasion Defining the relationship between ageing and cancer is a crucial but challenging task. Mice deficient in Zmpste24, a metalloproteinase mutated in human progeria and involved in nuclear prelamin A maturation, recapitulate multiple features of ageing. However, their short lifespan and serious cell-intrinsic and cell-extrinsic alterations restrict the application and interpretation of carcinogenesis protocols. Here we present Zmpste24 mosaic mice that lack these limitations. Zmpste24 mosaic mice develop normally and keep similar proportions of Zmpste24-deficient (prelamin A-accumulating) and Zmpste24-proficient (mature lamin A-containing) cells throughout life, revealing that cell-extrinsic mechanisms are preeminent for progeria development. Moreover, prelamin A accumulation does not impair tumour initiation and growth, but it decreases the incidence of infiltrating oral carcinomas. Accordingly, silencing of ZMPSTE24 reduces human cancer cell invasiveness. Our results support the potential of cell-based and systemic therapies for progeria and highlight ZMPSTE24 as a new anticancer target. Ageing and cancer are divergent consequences of the accumulation of molecular alterations with time. These changes activate cell senescence or apoptosis to prevent cancer, collaterally reducing fitness and regenerative potential [1] . The study of the ageing–cancer relationship is hampered by its complexity and duality, as ageing is caused by systemic and cellular alterations, and age is the main cancer risk factor. Disruption of the nuclear lamina, one of the cellular changes involved in natural ageing [2] , underlies different syndromes known as progeroid laminopathies [3] . Hutchinson-Gilford progeria syndrome, mandibuloacral dysplasia and restrictive dermopathy are caused by lamin A maturation defects due to mutations in the LMNA and the ZMPSTE24 loci, the latter encoding the metalloproteinase required for prelamin A processing [4] , [5] , [6] , [7] . Altered lamin A processing has been linked to senescence and upregulation of p53 targets, telomere erosion, defective DNA repair, increased autophagy, deregulated miRNA expression, epigenetic changes and overactivation of NF-κB signalling at the cellular level [8] , [9] , [10] , [11] , [12] , [13] , [14] . At the systemic level, prelamin A isoforms cause alterations in the somatotroph axis, changes in glucose and lipid metabolism, and induction of chronic inflammatory responses [14] , [15] . The wide and large effect of alterations of lamin A and its precursors on the pathways central for the control of cell viability and systemic homoeostasis processes, which are very frequently altered during oncogenesis, makes a potential link of nuclear lamins with cancer very plausible. However, the studies conducted so far have not established a clear connection [16] . Zmpste24 -deficient and Lmna- knock-in mice have been successfully used as models to study progerias and test potential treatments for them [17] , [18] , [19] . Unfortunately, these mice have important limitations that restrict the study of the relevance of prelamin A in cancer: their shortened lifespan (4 months) is not compatible with conventional tumour induction protocols, and their concomitant systemic and cellular abnormalities make it difficult to dissect the effects of prelamin A on tumour biology [4] . To circumvent these limitations, we describe herein the generation of a novel mosaic mouse model in which Zmpste24-deficient cells—accumulating prelamin A–and Zmpste24-proficient cells—expressing mature lamin A—coexist in similar proportions within the same individual, showing no overt phenotype and normal levels of systemic parameters typically altered in progeroid mice. Moreover, this model allowed us to analyse the effects of prelamin A on tumour establishment and progression in vivo . Zmpste24 mosaic mice display no progeroid phenotype We have generated a novel epigenetic-mosaic mouse model using recombination-mediated cassette exchange (RMCE) ( Fig. 1a and Supplementary Fig. S1a ), following a previously described strategy [20] . The mice in this study were Zmpste24 −/− Hprt Z24/+ females (hereafter ‘mosaic’): null for the autosomal Zmpste24 locus, but containing an extra copy of the Zmpste24 gene introduced at the Hprt locus of their X chromosome ( Fig. 1a and Supplementary Fig. S1a ). Because of random X inactivation, two types of cells should be present in them: those expressing Zmpste24 from their Hprt locus and those not expressing Zmpste24 at all. As controls, we generated Zmpste24 +/− Hprt Z24/+ female mice (hereafter ‘HT-control’), which are heterozygous for the autosomal Zmpste24 locus and thus would lack any deleterious phenotype [4] , and Zmpste24 −/− Hprt ΔZ24 /+ female mice (hereafter ‘KO-control’), which contain an insert in the Hprt locus ( ΔZ24 ) similar to the one in Zmpste24 −/− Hprt Z24/+ mice, but missing essential Zmpste24- coding sequences ( Fig. 1a and Supplementary Fig. S1b ). To facilitate the monitoring of X inactivation, we also introduced into the Hprt locus a CAGGS-DsRed reporter cassette in cis with the Zmpste24 and ΔZ24 inserts ( Supplementary Fig. S1a,c ). Mosaic, HT-control and KO-control mice were born at the expected Mendelian ratios. 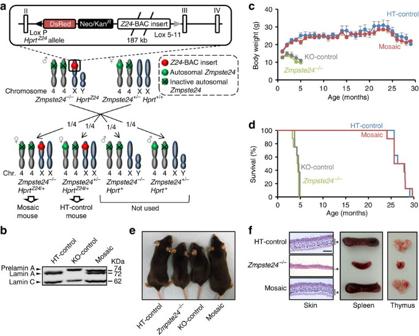Figure 1: Absence of progeroid phenotype in Zmpste24 mosaic mice. (a) Breeding scheme.Zmpste24−/−HprtZ24male mice were bred withZmpste24+/−Hprt+/+female mice to yield female offspring that were eitherZmpste24−/−HprtZ24/+(mosaic) orZmpste24+/−HprtZ24/+(HT-control). (b) Western blot analysis of lamins A and C from control and mosaic neonatal fibroblasts. Original immunoblots images are shown inSupplementary Fig. S7. (c) Body weight versus age of HT-control, KO-control,Zmpste24−/−and mosaic mice (n=5 per genotype). Error bars represent s.e.m. (d) Kaplan–Meier survival plot of mice with genotypes as inc(n=8 per genotype). (e) Photographs of 4-month-old HT-control,Zmpste24−/−, KO-control and mosaic mice. (f) Lack of progeroid features in skin, thymus and spleen from mosaic mice. Asterisk-labelled bars indicate the depth of the subcutaneous fat layer. Scale bar, 500 μm. Figure 1: Absence of progeroid phenotype in Zmpste24 mosaic mice. ( a ) Breeding scheme. Zmpste24 −/− Hprt Z24 male mice were bred with Zmpste24 +/− Hprt +/+ female mice to yield female offspring that were either Zmpste24 −/− Hprt Z24 /+ (mosaic) or Zmpste24 +/− Hprt Z24 /+ (HT-control). ( b ) Western blot analysis of lamins A and C from control and mosaic neonatal fibroblasts. Original immunoblots images are shown in Supplementary Fig. S7 . ( c ) Body weight versus age of HT-control, KO-control, Zmpste24 −/− and mosaic mice ( n =5 per genotype). Error bars represent s.e.m. ( d ) Kaplan–Meier survival plot of mice with genotypes as in c ( n =8 per genotype). ( e ) Photographs of 4-month-old HT-control, Zmpste24 −/− , KO-control and mosaic mice. ( f ) Lack of progeroid features in skin, thymus and spleen from mosaic mice. Asterisk-labelled bars indicate the depth of the subcutaneous fat layer. Scale bar, 500 μm. Full size image To ascertain the production of functional Zmpste24 metalloproteinase from the Zmpste24 gene at the Hprt locus, we obtained protein extracts from mosaic pups and performed lamin A and prelamin A western blot analysis. Although in the presence of autosomal Zmpste24 (HT-control) just lamin A was detected, and in its absence (KO-control) only prelamin A was observed, extracts from newborn ear mosaic fibroblasts contained lamin A and prelamin A, consistent with the co-existence of Zmpste24-deficient and -proficient cells ( Fig. 1b ). Interestingly, mosaic mice were phenotypically indistinguishable from wild-type or HT-controls, as they did not present the progeroid phenotypes and shortened lifespan of Zmpste24 −/− or KO-control mice ( Fig. 1c–f ). These results indicate that mosaic Zmpste24 complementation generates lamin A-expressing cells that elicit reversion of the progeroid phenotype induced by prelamin A in Zmpste24 -deficient mice. Zmpste24-deficient and -proficient cells thrive equally To evaluate the persistence of prelamin A-expressing cells in mosaic mice, we performed DsRed fluorescence analysis of different organs. Prelamin A-containing cells display replicative defects in Zmpste24 -deficient mice [11] . If this was the case in mosaic mice, we should detect a replacement of cells not expressing Zmpste24 by those expressing this metalloproteinase. Interestingly, all organs studied from 1-year-old mosaic mice, double the maximum lifespan of Zmpste24 −/− mice, contained fluorescent (DsRed-positive) and non-fluorescent cells ( Fig. 2a ). Furthermore, immunohistochemical labelling of DsRed and prelamin A in hearts from mosaic mice confirmed that DsRed-expressing cells contained Zmpste24 that was able to process prelamin A, whereas this lamin A precursor was accumulated in DsRed-negative cells ( Fig. 2b ). To analyse whether cell substitution occurred with age, we dissected tissues from 2-month-, 1-year- and 2-year-old mice and measured their DsRed fluorescence. We did not detect significant changes in the intensity of red fluorescence in any organ except for the heart, where a consistent increase of DsRed signal was apparent ( Fig. 2c ). However, this increase was also detected in HT-control and in Zmpste24 +/− Hprt ΔZ24 /+ animals, which only contain Zmpste24-proficient cells, ruling out the possibility that it was related to the effects of prelamin A ( Supplementary Fig. S2 ). Then, as red fluorescence is an indirect reporter of Zmpste24 expression, we confirmed our results by immunoblotting of Zmpste24, lamin A and prelamin A in tissues from 4-, 12- and 24-month-old mice ( Fig. 2d and Supplementary Fig. S3 ). Consistently, no significant changes on the levels of these proteins were detected. 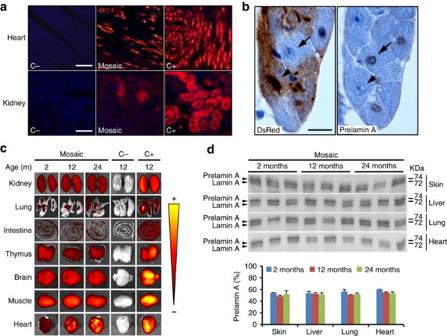Figure 2: Zmpste24-deficient cells are detected throughout lifespan of mosaic mice. (a) Fluorescence microscopy of DsRed-expressing cells in tissues fromZmpste24+/+Hprt+/+(C−), mosaic andZmpste24+/−HprtZ24/Z24(C+) mice. Scale bars, 100 μm (heart) and 50 μm (kidney). (b) Immunohistochemical analysis of DsRed (left) and prelamin A (right) in mosaic hearts. Arrows correspond to a Zmpste24-deficient cell (DsRed−, prelamin A+), whereas arrowheads point to aZmpste24-proficient cell (DsRed+, prelamin A−). Scale bar, 10 μm. (c) DsRed fluorescent signal detection by anIn VivoImaging System in whole organs from mosaic mice at different ages, compared with the same organs from 1-year-oldZmpste24+/+Hprt+/+(C−) andZmpste24+/−HprtZ24/Z24(C+) mice. For comparison with DsRed signal in hearts from HT-control andZmpste24+/−HprtΔZ24/+mice, seeSupplementary Fig. S2. (d) Western blot analysis of prelamin A and lamin A from skin, liver, lung and heart of 2-, 12- and 24-month-old mosaic mice. A densitometry analysis of the immunoblots is also shown. Error bars represent s.e.m.n=3. Figure 2: Zmpste24-deficient cells are detected throughout lifespan of mosaic mice. ( a ) Fluorescence microscopy of DsRed-expressing cells in tissues from Zmpste24 +/+ Hprt +/+ (C−), mosaic and Zmpste24 +/− Hprt Z24 /Z24 (C+) mice. Scale bars, 100 μm (heart) and 50 μm (kidney). ( b ) Immunohistochemical analysis of DsRed (left) and prelamin A (right) in mosaic hearts. Arrows correspond to a Zmpste24-deficient cell (DsRed−, prelamin A+), whereas arrowheads point to a Zmpste24 -proficient cell (DsRed+, prelamin A−). Scale bar, 10 μm. ( c ) DsRed fluorescent signal detection by an In Vivo Imaging System in whole organs from mosaic mice at different ages, compared with the same organs from 1-year-old Zmpste24 +/+ Hprt +/+ (C−) and Zmpste24 +/− Hprt Z24 /Z24 (C+) mice. For comparison with DsRed signal in hearts from HT-control and Zmpste24 +/− Hprt ΔZ24 /+ mice, see Supplementary Fig. S2 . ( d ) Western blot analysis of prelamin A and lamin A from skin, liver, lung and heart of 2-, 12- and 24-month-old mosaic mice. A densitometry analysis of the immunoblots is also shown. Error bars represent s.e.m. n =3. Full size image To finely measure the proportions of Zmpste24-deficient and -proficient cells in different tissues with age, we pyrosequenced bisulphite-modified DNA. This approach allowed us to detect methylation of specific CpG dinucleotides in the Zmpste24 promoter located at the Hprt locus, which shows maximum levels of methylation in the inactive X chromosome ( Fig. 3a ). To set the maximum methylation value, we analysed two lines of Zmpste24-deficient ear fibroblasts isolated from mosaic mice by random drift during serial passages in culture ( Fig. 3a ). These cells only produce prelamin A, thereby representing the highest level of methylation observable. CpG 3 and CpG 4 dinucleotides showed methylation values consistently high in these Zmpste24-deficient cells. We focused on CpG 3 and set the 100% methylation level as the average value obtained for this dinucleotide in Zmpste24-deficient cells. As expected, CpG 3 methylation in all tissues from wild-type mice was negligible ( Fig. 3a ). We then analysed tissues from mosaic mice and HT-control mice ( Fig. 3b ). If substitution of Zmpste24-deficient cells by Zmpste24-proficient cells occurred, the percentage of methylation in the Zmpste24 promoter should decrease with age in the mosaic mice. However, methylation levels did not decrease significantly with time in mosaic tissues and remained similar to the values obtained in HT-control tissues between 2 months and 2 years, including the heart ( Fig. 3b ). 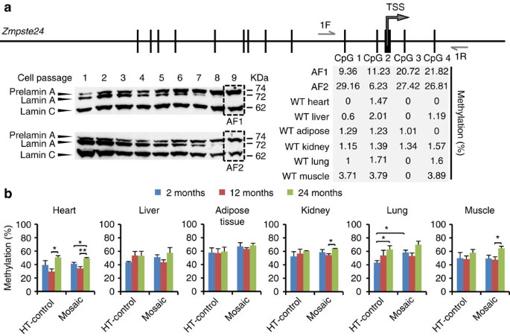Figure 3: Mosaic mice keep similar proportions of Zmpste24-deficient and -proficient cells at all ages. (a) Bisulphite pyrosequencing strategy to quantify the relative proportion of Zmpste24-deficient and -proficient cells. Four CpG sites around theZmpste24promoter were analysed in DNA from Zmpste24-deficient AFs isolated from mosaic mice (AF1 and AF2) and in DNA from six wild-type tissues (heart, liver, adipose tissue, kidney, lung and muscle). Western blots show the progressive loss of mature lamin A and accumulation of prelamin A with serial passages of AF1 and AF2 cells, until only prelamin A is detected (dashed rectangles). The percent methylation of CpG sites is depicted for each of the cell populations. CpG 3 was subsequently used because of its low levels of methylation in wild-type tissues and consistent high values in the isolated fibroblasts. 1F and 1R indicate the positions of the oligonucleotides used (for sequences, seeSupplementary Table S4). TSS,Zmpste24transcription start site. (b) QuantitativeZmpste24methylation analysis by pyrosequencing in different organs from 2-, 12- and 24-month-old mosaic and HT-control mice (n≥3). Error bars represent s.e.m. *P<0.05; **P<0.01; and two-tailed Student’st-test. Figure 3: Mosaic mice keep similar proportions of Zmpste24-deficient and -proficient cells at all ages. ( a ) Bisulphite pyrosequencing strategy to quantify the relative proportion of Zmpste24-deficient and -proficient cells. Four CpG sites around the Zmpste24 promoter were analysed in DNA from Zmpste24-deficient AFs isolated from mosaic mice (AF1 and AF2) and in DNA from six wild-type tissues (heart, liver, adipose tissue, kidney, lung and muscle). Western blots show the progressive loss of mature lamin A and accumulation of prelamin A with serial passages of AF1 and AF2 cells, until only prelamin A is detected (dashed rectangles). The percent methylation of CpG sites is depicted for each of the cell populations. CpG 3 was subsequently used because of its low levels of methylation in wild-type tissues and consistent high values in the isolated fibroblasts. 1F and 1R indicate the positions of the oligonucleotides used (for sequences, see Supplementary Table S4 ). TSS, Zmpste24 transcription start site. ( b ) Quantitative Zmpste24 methylation analysis by pyrosequencing in different organs from 2-, 12- and 24-month-old mosaic and HT-control mice ( n ≥3). Error bars represent s.e.m. * P <0.05; ** P <0.01; and two-tailed Student’s t -test. Full size image To further explore these in vivo observations, we studied whether the presence of wild-type cells is able to rescue the phenotype of Zmpste24 -deficient fibroblasts in vitro . The growth dynamics of co-cultures of adult fibroblasts (AFs) explanted from wild-type and Zmpste24 -knockout mice closely resembled that of wild-type AFs, suggesting that Zmpste24 -deficient AFs proliferate better in the presence of wild-type cells ( Supplementary Fig. S4a ). To analyse whether, as previously reported for LMNAΔ9 mouse AFs [21] , the presence of extracellular matrix (ECM) alone was able to rescue the proliferative ability of Zmpste24 -deficient AFs, we cultured them on ECM previously deposited by wild-type or Zmpste24 -deficient AFs. Interestingly, both types of ECM improved the replicative capacity of Zmpste24 -deficient AFs, suggesting that an ECM production deficit, and not the lack of specific components of the ECM, underlies the reduced proliferative ability of Zmpste24 -deficient cells in vitro ( Supplementary Fig. S4b ). Taken together, these results indicate that prelamin A accumulation does not represent a selective disadvantage for cells of mosaic mice, where Zmpste24-deficient and -proficient cells coexist in similar proportions, and suggest that ECM-mediated mechanisms contribute to the reversal of the phenotype of Zmpste24 -deficient cells. Progeria markers are rescued in mosaics Because p53-target genes are overexpressed in hearts from Zmpste24 −/− mice [11] , we analysed cardiac p21, Atf3 and Igfbp3 mRNA levels in mosaic mice. Although Zmpste24 -deficient hearts showed overexpression of these three p53-target mRNAs, the levels of these transcripts were normal in mosaic hearts ( Fig. 4a ). To further explore this observation, we used DsRed labelling to separate Zmpste24-deficient cells from Zmpste24-proficient cells by microdissection of mosaic hearts. Interestingly, p21 and Igfbp3 levels were not significantly different in Zmpste24-deficient and -proficient cardiomyocytes from the same mosaic mouse ( Fig. 4b ). Together, these results indicate that the upregulation of p53-target transcripts in Zmpste24 -deficient mice is not a direct consequence of prelamin A accumulation in each cell, but likely secondary to the progressive organismal deterioration of these animals. We next analysed the levels of biochemical markers and hormones deregulated in the complete absence of Zmpste24 (refs 11 , 15 ). IGF1, glucose and major urinary protein levels were normal in mosaic mice ( Fig. 4c,d ). Thus, these animals appear healthy, despite containing a high proportion of prelamin A-expressing, Zmpste24-deficient cells. All these observations further support the idea that cell-extrinsic mechanisms are preeminent in the onset and development of prelamin A-induced progeria. 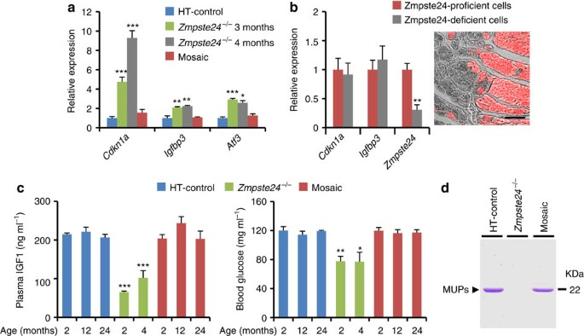Figure 4: Rescue of molecular and systemic progeria markers in mosaic mice. (a) Transcriptional qPCR analysis of p53-target genes (Cdkn1a,Igfbp3andAtf3) in hearts from 6-month-old HT-control mice, 3-month- and 4-month-oldZmpste24−/−and 6-month-old mosaic mice. Data are shown as fold-change values as compared with HT-controls (n≥3). (b) Expression ofCdkn1a,Igfbp3andZmpste24in microdissected DsRed fluorescent and negative cells from 6-month-old mosaic hearts (n=3). A fluorescence photomicrograph of DsRed-positive (red) and -negative (grey) heart areas, representative of those used for microdissection, is shown on the right. Scale bar, 100 μm. (c) Plasma levels of IGF1 and blood glucose concentration in HT-control,Zmpste24−/−and mosaic mice of the indicated age (n≥3). In (a–c), error bars represent s.e.m. *P<0.05; **P<0.01; ***P<0.001; and two-tailed Student’st-test. (d) Representative picture of SDS–PAGE analysis of major urinary proteins (MUPs) content in urine from mice of each of the indicated genotypes. Figure 4: Rescue of molecular and systemic progeria markers in mosaic mice. ( a ) Transcriptional qPCR analysis of p53-target genes ( Cdkn1a , Igfbp3 and Atf3 ) in hearts from 6-month-old HT-control mice, 3-month- and 4-month-old Zmpste24 −/− and 6-month-old mosaic mice. Data are shown as fold-change values as compared with HT-controls ( n ≥3). ( b ) Expression of Cdkn1a , Igfbp3 and Zmpste24 in microdissected DsRed fluorescent and negative cells from 6-month-old mosaic hearts ( n =3). A fluorescence photomicrograph of DsRed-positive (red) and -negative (grey) heart areas, representative of those used for microdissection, is shown on the right. Scale bar, 100 μm. ( c ) Plasma levels of IGF1 and blood glucose concentration in HT-control, Zmpste24 −/− and mosaic mice of the indicated age ( n ≥3). In ( a – c ), error bars represent s.e.m. * P <0.05; ** P <0.01; *** P <0.001; and two-tailed Student’s t -test. ( d ) Representative picture of SDS–PAGE analysis of major urinary proteins (MUPs) content in urine from mice of each of the indicated genotypes. Full size image Prelamin A accumulation does not affect tumour initiation As Zmpste24 mosaic mice contain prelamin A-expressing cells in a normal environment, we used them to evaluate the potential role of A-type lamins in cancer. To compare the tumour initiation potential of prelamin A-expressing cells and normal lamin A-expressing cells, we performed two protocols: topical 7,12-dimethylbenz[a]anthracene (DMBA)–12-o-tetradecanoylphorbol-13-acetate (TPA) application for the induction of skin papillomas [22] and urethane injection for the generation of lung adenomas [23] . We did not detect differences in tumour susceptibility between HT-control and mosaic mice or in the number of tumours expressing or lacking prelamin A in the latter animals ( Supplementary Fig. S5a–c ). Consistent with these observations, no significant differences in Ki67 staining were detectable between prelamin A-positive and -negative tumours ( Supplementary Fig. S5d ). Thus, prelamin A does not affect the susceptibility of epithelial cells from the skin or lung to neoplasia. Prelamin A accumulation prevents cancer invasion To test whether prelamin A could have a role in cancer progression, we performed an additional carcinogenesis protocol based on the administration of 4-nitroquinoline 1-oxide (4-NQO) in drinking water to induce squamous cell carcinomas of the upper digestive tract [24] . This protocol produced a wide spectrum of neoplastic lesions, from benign papillomas to infiltrating carcinomas. In agreement with the above results, no differences were observed in premalignant lesions ( Fig. 5a ). However, the proportion of mosaic mice affected by infiltrating carcinomas of the oral cavity was significantly reduced, as compared with HT-controls ( Fig. 5a ). Moreover, the proportion of oral infiltrating carcinomas with respect to all carcinomas (carcinomas in situ plus infiltrating carcinomas) was also strikingly lower in the mosaic mice ( Fig. 5b ). Interestingly, although the numbers of carcinomas in situ expressing and not expressing prelamin A by immunohistochemistry were comparable in mosaic mice ( Fig. 5c ), the only two infiltrating carcinomas observed in these animals lacked prelamin A staining ( Fig. 5d ). 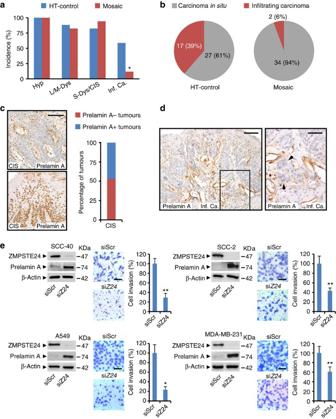Figure 5: Prelamin A accumulation prevents cancer invasion. (a) Percentage of HT-control (n=17) and mosaic (n=17) mice affected by oral lesions with the indicated histology. CIS, carcinomain situ; Hyp, hyperplasia; Inf. Ca., infiltrating carcinoma; L/M-Dys, light/moderate dysplasia; S-Dys, severe dysplasia. (b) Number and proportion ofin situand infiltrating oral carcinomas in each group. (c) Representative photomicrographs of positive (bottom) and negative (top) prelamin A staining in oral CIS from mosaic mice. The percentage of prelamin A-positive and -negative CIS is plotted. A total of 17 CIS were analysed by prelamin A immunohistochemistry. Scale bar, 100 μm. (d) Representative photomicrographs of a prelamin A-negative infiltrating carcinoma from a mosaic mouse. Arrowheads point at nests of invasive cancer cells. Scale bars, 100 μm (left panel) and 50 μm (right panel). (e) Effect ofZMPSTE24silencing on the invasiveness of SCC-40, SCC-2, A549 and MDA-MB-231 cancer cell lines. Left panels: western blots showing the accumulation of prelamin A uponZMPSTE24(siZ24)versus scrambled (siScr) silencing. Right panels: representative pictures and average number of invasiveZMPSTE24-interfered and scrambled-treated cells. The assays were carried out at least in triplicate, and results are expressed as mean±s.e.m. *P<0.05; **P<0.01; and Fisher’s exact test. Scale bars, 100 μm. Figure 5: Prelamin A accumulation prevents cancer invasion. ( a ) Percentage of HT-control ( n =17) and mosaic ( n =17) mice affected by oral lesions with the indicated histology. CIS, carcinoma in situ ; Hyp, hyperplasia; Inf. Ca., infiltrating carcinoma; L/M-Dys, light/moderate dysplasia; S-Dys, severe dysplasia. ( b ) Number and proportion of in situ and infiltrating oral carcinomas in each group. ( c ) Representative photomicrographs of positive (bottom) and negative (top) prelamin A staining in oral CIS from mosaic mice. The percentage of prelamin A-positive and -negative CIS is plotted. A total of 17 CIS were analysed by prelamin A immunohistochemistry. Scale bar, 100 μm. ( d ) Representative photomicrographs of a prelamin A-negative infiltrating carcinoma from a mosaic mouse. Arrowheads point at nests of invasive cancer cells. Scale bars, 100 μm (left panel) and 50 μm (right panel). ( e ) Effect of ZMPSTE24 silencing on the invasiveness of SCC-40, SCC-2, A549 and MDA-MB-231 cancer cell lines. Left panels: western blots showing the accumulation of prelamin A upon ZMPSTE24 (si Z24) versus scrambled (siScr) silencing. Right panels: representative pictures and average number of invasive ZMPSTE24 -interfered and scrambled-treated cells. The assays were carried out at least in triplicate, and results are expressed as mean±s.e.m. * P <0.05; ** P <0.01; and Fisher’s exact test. Scale bars, 100 μm. Full size image To explore the mechanistic basis of this observation in a human cancer context, we used small interfering RNAs (siRNAs) to silence ZMPSTE24 in cell lines from human oral infiltrating carcinomas (SCC-40 and SCC-2) and compared their RNA expression profiles with those of mock-treated cells. ZMPSTE24 silencing produced prelamin A accumulation and induced relevant changes in gene expression. Interestingly, gene set enrichment analysis revealed that among the pathways most significantly altered in ZMPSTE24- silenced SCC-40 and SCC-2 cells are those involved in ECM composition and in cell–ECM interactions ( Supplementary Tables S1–S3 ). This observation, together with the well-established relationship between ECM and cancer cell invasiveness, prompted us to test whether prelamin A accumulation also affected the invasive properties of these cancer cell lines. Consistent with our in vivo results, in vitro invasion assays with ZMPSTE24- silenced SCC-40 and SCC-2 cells showed that the accumulation of prelamin A caused a significant decrease of their invasive potential ( Fig. 5e ). To study whether this effect was specific to oral cancer, we analysed breast (MDA-MB-231) and lung (A549) cancer cells, observing a reduction in their invasive ability in the presence of prelamin A ( Fig. 5e ). Genome-wide expression profiles of these cells upon ZMPSTE24 silencing also pointed to the pathways involved in the synthesis of precursors of ECM components as the most significant commonly altered molecular routes ( Supplementary Table S1 ). In addition, all four cell lines studied showed significant changes in expression of main components of the ECM–receptor interaction pathways, such as ITGA5 , CD47 or DAG1 ( Supplementary Table S2 ). Thus, ZMPSTE24 silencing in oral, breast and lung cancer cell lines causes prelamin A accumulation and rewiring of the ECM-related cellular pathways, which could account for their reduced invasive potential. Interestingly, all four ZMPSTE24 -silenced cancer cell lines that were analysed showed alterations in routes involved in proteoglycan synthesis (chondroitin sulphate and/or heparan sulphate (HS)) ( Supplementary Tables S1,S3 ), showing expression changes indicative of increased production of oversulfated forms of both ECM components. Human lifespan extension is rising the incidence of pathologies associated with age, of which cancer is the second most lethal, only after cardiovascular disease [25] . Age is the main risk factor for cancer incidence, but the links between ageing and cancer remain difficult to define because of the complex relationship between both processes [26] . Besides causing accelerated ageing syndromes, immature lamin A forms accumulate with advancing age in non-progeroid cells and have been linked to the activation of tumour-suppressor mechanisms [2] , [11] . Accordingly, one potential role for prelamin A would be the protection against cancer. Because of their short lifespan, mouse models of progeroid laminopathies are not suitable for the analysis of the effects of lamin A precursors on cancer. To circumvent this limitation, we have created a novel mosaic mouse model containing prelamin A-accumulating and normal cells. These mice do not suffer from premature death and, therefore, are suitable to study the effects of this lamin A precursor on tumour initiation and progression. Our thorough analysis of mosaic mice has revealed that prelamin A accumulation does not represent a selective disadvantage for cells, demonstrating that cell-extrinsic mechanisms are preeminent in progeria pathogenesis. This finding was unexpected, as abnormal prelamin A processing causes defects in essential cell pathways [9] , [10] , [11] , [27] , [28] , [29] , [30] , [31] , [32] . In line with our observations, Song et al. [33] have recently shown that exposure of progeroid Zmpste24 -deficient muscular-derived stem/progenitor cells to wild-type muscular-derived stem/progenitor cells rescues their myogenic differentiation defect in vitro . Even in the light of this observation, the complete absence of progeroid features in our mosaic mice is a remarkable and encouraging finding. Our results suggest that the positive effects of Zmpste24-proficient cells on Zmpste24-deficient cells are mediated by a combination of structural and diffusible factors. Thus, the replicative defects shown by Zmpste24 -deficient AFs grown in vitro are rescued by the presence of ECM. This observation recapitulates the results previously obtained with LMNAΔ9 mouse AFs [21] . In addition, circulating levels of systemic factors such as IGF1 are restored in mosaic mice. Although, from our observations, we cannot distinguish whether the normal levels of IGF1 are responsible for the lack of progeroid phenotype or a consequence of it in mosaic mice, the positive effect of the administration of this hormone to Zmpste24 -deficient mice supports the existence of a causative role for IGF1 on the prevention of progeria [15] . Moreover, our findings highlight the potential relevance of both systemic and cell-based or gene-correction treatments for progeroid syndromes and pathologies associated with normal ageing [18] , [34] . In this regard, parabiosis experiments, in which the circulatory systems of young and old mice are artificially connected, have already shown the potential of systemic factors to prevent certain characteristics of natural ageing [35] , [36] . One of these, the TGF-β superfamily member GDF11, has been recently identified as a circulating factor in young mice that declines with age and is able to reverse age-related cardiac hypertrophy when administered to old mice [35] . On the other hand, the generation of genetically corrected induced pluripotent stem cells from Hutchinson-Gilford progeria syndrome fibroblasts, or the feasibility to perform in vivo genomic editing, creates novel treatment options for these pathologies that need to be further explored [37] , [38] , [39] , [40] . Our results, showing that full reversion of the progeroid phenotype is compatible with the persistence of a high proportion of prelamin A-expressing cells, reinforce the potential held by gene-correction and cell-based therapeutic approaches to tackle these dramatic progeroid syndromes. Cancer induction experiments performed in mosaic mice indicate that prelamin A does not affect tumour initiation, but it prevents cancer invasion. This was confirmed in human oral, lung and breast cancer cell lines, suggesting that cancer invasion might display non-oncogenic addiction to the ZMPSTE24 metalloproteinase [41] . Molecular surveillance of the acquisition of invasive properties constitutes a plausible cancer control checkpoint. Thus, although the loss of p53 has no effect on the number of mutant- Kras -induced lung tumours or mutant- Braf -induced colorectal adenomas, its presence prevents the progression of benign adenomas into adenocarcinomas [42] , [43] , [44] . The accumulation of immature lamin A isoforms might constitute one of those mechanisms that could become stronger with time to compensate for the increased cancer risk inherent to ageing [2] . The observed expression changes in the pathways involved in ECM composition upon ZMPSTE24 silencing in human cancer cell lines indicate that prelamin A might exert this protective effect through a cell-extrinsic mechanism. Actually, the ECM and its interactors are main characters of cancer invasion [45] . Although increased levels of proteoglycans have been linked to enhanced invasion, recent work has shown that both chondroitin sulphate and HS can exert different roles depending on their specific modifications (such as oversulfation) and microenvironment [46] , [47] . Moreover, synthetic HS mimetics have been proposed as anticancer agents able to inhibit tumour progression and metastasis, opening the possibility that specific natural HS isoforms might have similar anticancer roles [48] . The potential cell-extrinsic effect of prelamin A accumulation on prevention of cancer cell invasion is supported by the fact that the proportion of carcinomas displaying invasive properties in mosaic mice (6%) is far below half of that observed in HT-controls (39%). On the other hand, the only two oral infiltrating carcinomas observed in mosaic mice lacked prelamin A expression, and this would be consistent with a cell-autonomous effect of prelamin A on invasion prevention. Further work involving prelamin A expression analysis on a much larger number of infiltrating carcinomas will be required to clarify this issue. In summary, we have developed a novel mosaic mouse model constituted by prelamin A-accumulating cells and mature lamin A-expressing cells in similar proportions, which shows no overt phenotype. Besides representing a useful tool for the study of the relevance of prelamin A in cancer initiation and progression, the molecular and cellular characterization of these mice highlights the importance of cell-extrinsic mechanisms for the establishment of laminopathy-based progerias. Moreover, it suggests that cell/gene therapies and supplementation of systemic factors hold great potential to tackle these degenerative diseases. These approaches could be combined with the pharmacological strategies already proven to work in animal models that are currently being evaluated in clinical trials [19] . In addition, the role of prelamin A against cancer invasion suggests that ZMPSTE24 metalloproteinase could be an attractive new target for cancer therapy. Generation of the Hprt Z24 allele The RP23-227I2 BAC clone was modified by the introduction of a pgk/EM7-Neo/KanR-CAGGS-DsRed cassette, permitting positive selection in bacteria (with kanamycin) and eukaryotic cells (with G418) and controlling the expression of the fluorescent protein DsRed. For the generation of the pgk/EM7-Neo/Kan R -CAGGS-DsRed cassette, elements from three different plasmids were used: pCEI1, MG1 and pDsRed-Monomer-N1. pCEI1 was described in the original paper introducing the RMCE technique [20] . This plasmid contains the Neo/KanR gene controlled by the pgk/EM7 promoter and flanked by mini arms of homology for the sacBII gene, which permit insertion of the resistance cassette in the BAC by homologous recombination in bacteria. The MG1 plasmid was created by H.M.P. and contains the CAGGS promoter from the pCAGGS vector [49] , but with a more versatile cloning site. The pDsRed-Monomer-N1 plasmid (Clontech) contains the cDNA for the Monomer-N1 version of the red fluorescent protein DsRed. First, the Not I site from pDsRed-Monomer-N1 was destroyed. For that purpose, this plasmid was linearized by Not I digestion, the protruding ends were blunted with Klenow and the plasmid was religated and transformed in competent Escherichia coli cells to generate pDsRed-Monomer-N1- Not I-Dest. After that, the MG1 plasmid was digested with Afl II, a 1,759-bp fragment containing the CAGGS promoter was isolated and blunted with Klenow, and that fragment was cloned into pDsRed-Monomer-N1- Not I-Dest that had been previously linearized with Hin dIII and Eco RI, blunted with Klenow and dephosphorylated, to generate the pCAGGS-DsRed-Monomer-N1 plasmid. Finally, pCAGGS-DsRed-Monomer-N1 was digested with Hin dIII and Afl II to isolate a 2,750-bp fragment containing the CAGGS-DsRed-Monomer-N1 cassette, which was blunted with Klenow and cloned into pCEI1, previously linearized with Bam H1, blunted with Klenow and dephosphorylated. This produced the pCEI1-CAGGS-DsRed-Monomer-N1 plasmid. This plasmid can be used to introduce kanamycin/G418-resistance ability and DsRed expression into any BAC containing the sacBII gene. This vector was linearized with Not I and electroporated into electrocompetent EL350 cells that had been previously transformed with the RP23-227I2 BAC according to previously described protocols [50] . To isolate recombinant clones containing the BAC modified with the pgk/EM7-Neo/Kan R -CAGGS-DsRed cassette, chloramphenicol and kanamycin selection was applied (the backbone from the BAC provides chloramphenicol resistance and the pgk/EM7-Neo/Kan R -CAGGS-DsRed cassette provides kanamycin resistance). The identity of the BAC was checked by digestion with restriction enzymes, BAC DNA was isolated from a positive EL350 clone, and it was retransformed into DH10B bacteria for large-scale isolation of the modified BAC, as previously described [20] . The Hprt Z24 allele was generated following a strategy very similar to that previously described [20] . Analysis of BAC insert integrity by array CGH Four recombinant embryonic stem (ES) cell clones (A1, A3, A10 and A12) were selected for detailed analysis of BAC insert integrity, as partial insert deletions have been described in ES cell clones generated by RMCE [20] . Insert integrity was analysed using a custom Roche Nimblegen CGH 4-plex Array. Each of the four subfields of the array contained two different regions: a high-resolution region, made of 45,000 probes evenly distributed between genomic coordinates 120,627,332 and 120,942,331 of mouse chromosome 4 excluding repetitive DNA regions (1 probe every 4 bp), and a low-resolution region, consisting of 25,000 probes homogenously scattered along the whole mouse genome (one probe every 100 kb). The high-resolution region spans the whole BAC insert, plus two additional 64,171-bp long sequences, corresponding to the mouse chromosome 4 regions flanking the sequence contained in the BAC insert at its 5′ and 3′ ends. The array-CGH results were analysed with SignalMap, which permitted the detection of a 38,200-bp deletion in clone A2, corresponding approximately to coordinates 120,742,750–120,780,950 of mouse chromosome 4, and thus containing the first seven exons of Zmpste24 . No alterations were observed in inserts from clones A1, A3 and A12 ( Supplementary Fig. S1b ). Mouse strains Animal experiments were conducted in accordance with the guidelines of the Committee on Animal Experimentation of the University of Oviedo. Mutant mice deficient in the Zmpste24 metalloproteinase have been described previously [4] . Hprt Z24 and Hprt ΔZ24 mice were obtained from A3 and A2 ES cell clones, respectively ( Supplementary Fig. S1b ). Zmpste24 −/− Hprt Z24/+ mice were obtained by crossing Zmpste24 +/− male mice with Hprt Z24/+ female mice to produce Zmpste24 +/− Hprt Z24 males and Zmpste24 +/− Hprt Z24/+ females. These mice were backcrossed with Zmpste24 +/− mice to produce Zmpste24 −/− Hprt Z24 male mice. Those males were subsequently backcrossed with Zmpste24 +/− mice to produce mosaics and HT-controls. Zmpste24 −/− Hprt ΔZ24/+ mice were obtained by crossing Zmpste24 +/− male mice with Hprt ΔZ24/+ female mice to get Zmpste24 +/− Hprt ΔZ24 male mice and Zmpste24 +/− Hprt ΔZ24/+ female mice, which were backcrossed with Zmpste24 +/− mice to obtain KO-controls. Mosaic mice were genotyped by a combination of conventional and quantitative PCR ( Supplementary Fig. S6 ). In Vivo imaging system For whole-organ DsRed imaging, fresh organs were placed on black cards and analysed for fluorescence using the in vivo imaging system (Xenogen). DsRed was excited at 570 nm and detected at 600 nm. Data were collected and analysed using Living Image software v3.1 (Xenogen). Bisulphite pyrosequencing assays Sodium bisulphite modification of 0.5 μg genomic DNA isolated from various tissues was carried out with the EZ DNA Methylation Kit following the manufacturer’s protocol. Bisulphite-treated DNA was eluted in 15 μl, and 2 μl were used as template for each PCR. The set of primers for PCR amplification and sequencing was designed using a specific software pack (PyroMark assay design version 2.0.01.15). Primers were designed to hybridize with CpG-free sites to ensure methylation-independent amplification (see Supplementary Table S4 ). PCR was performed with biotinylated primers to facilitate the conversion of the PCR product to single-stranded DNA templates. Vacuum Prep Tool (Biotage, Sweden) was used to prepare single-stranded PCR products according to the manufacturer’s instructions. Pyrosequencing reactions and methylation quantification were performed in a PyroMark Q24 System version 2.0.6 (Qiagen). Graphs of methylation values show bars identifying CpG sites with values ranging from 0 to 100%. Blood and plasma parameters Mice were fasted for 5 h to avoid alterations in blood parameters due to food intake previous to measurements. Blood glucose was measured with an Accu-Chek glucometer (Roche Diagnostics) using blood from the tail vein. For other parameters, blood was extracted directly from the mandibular sinus after anesthetizing mice with isoflurane. To obtain plasma, blood was centrifuged immediately after collection at × 3,000 g and 4 °C, and the supernatant was collected and stored at −80 °C until analysis. Plasma IGF1 concentration was determined using the R&D Systems Quantikine ELISA kit, according to the manufacturer’s instructions. Carcinogenesis protocols and analysis of tumours Mice were all female littermates aged 6–8 weeks at the start of tumour induction protocols. For the generation of skin tumours, mice were shaved and treated with a single dose of DMBA (Sigma; 25 μg in 200 μl acetone). Subsequently, mice were treated twice weekly with TPA (Sigma; 200 μl of 10 −4 M solution in acetone) for 12 consecutive weeks. Mice were killed 17 weeks after the start of treatment, and tumours were either snap-frozen in liquid nitrogen or fixed and processed for histological studies. For the generation of lung tumours, mice were intraperitoneally injected with 1 g kg −1 of urethane (Sigma) once a week for 8 consecutive weeks. Mice were killed at 28 weeks following the initial urethane injection. Then, lungs were fixed in 4% paraformaldehyde, paraffin-embedded, sectioned and stained with haematoxylin and eosin for morphological examination. For the generation of upper digestive tract tumours, a stock solution of the carcinogen 4-NQO (Sigma) was prepared weekly in propylene glycol at 5 mg ml −1 and stored at 4 °C. Mice were provided drinking water containing 4-NQO (100 μg ml −1 ) ad libitum during the treatment. After a 20-week carcinogen treatment, mice were kept alive for 2 more weeks and killed. Blocks containing the tongues together with the lower mandibles of mice were dissected immediately, fixed in 4% paraformaldehyde, decalcified if necessary, paraffin-embedded, sectioned and stained with haematoxylin and eosin for pathological examination. Gene-silencing and invasion assays For gene-silencing experiments, cells were transfected with 50 nM final concentration of ZMPSTE24 or negative-control Stealth RNAi siRNAs (Life Technologies; catalogue numbers: HSS115696 and HSS115697 for human ZMPSTE24 and 12935-300 for negative-control scramble siRNA) using Lipofectamine RNAi Max (Life Technologies) in Opti-MEM I Reduced Serum Medium without serum (Gibco) following the manufacturer’s instructions. In vitro invasion potential was evaluated using 24-well Matrigel-coated invasion chambers with an 8 μm pore size (BD Biosciences). For SCC-40 and A549 cell lines, 5 × 10 4 and 3 × 10 4 cells, respectively, were allowed to invade for 48 h using 10% fetal bovine serum as chemoattractant. In the case of SCC-2 and MDA-MB-231 cells, the invasion ability of 2.5 × 10 4 cells was evaluated for 24 h, using 5% fetal bovine serum as chemoattractant. Cells that reached the lower surface were stained with crystal violet and counted under the microscope. Gene expression arrays Global RNA expression profiling was done using Illumina HumanHT-12 version 4 beadchip. Data were quantile normalized and analysed using the bioconductor ( http://www.bioconductor.org/ ), lumi ( http://www.bioconductor.org/packages/2.0/bioc/html/lumi.html ) and limma packages, and then P -value was adjusted for multiple testing. Gene set enrichment analysis Gene set enrichment analysis (GSEA) was performed as described [51] . For data analysis, we used GSEA release 3.4 and MSigDB release 3.0 ( http://www.broadinstitute.org/gsea/index.jsp ). Weighted enrichment scores were calculated with gene expression lists ranked by signal to-noise ratio. The number of permutations was set to 1,000. Analyses were focused on curated gene sets from the canonical pathway subcollection. Accession codes : RNA expression data have been deposited in the Gene Expression Omnibus repository under accession code GSE41799 . How to cite this article: de la Rosa, J. et al. Prelamin A causes progeria through cell-extrinsic mechanisms and prevents cancer invasion. Nat. Commun. 4:2268 doi: 10.1038/ncomms3268 (2013).